Phytochrome B and REVEILLE1/2-mediated signalling controls seed dormancy and germination inArabidopsis Seeds maintain a dormant state to withstand adverse conditions and germinate when conditions become favourable to give rise to a new generation of flowering plants. Seed dormancy and germination are tightly controlled by internal and external signals. Although phytochrome photoreceptors are proposed to regulate primary seed dormancy, the underlying molecular mechanism remains elusive. Here we show that the REVEILLE1 (RVE1) and RVE2 transcription factors promote primary seed dormancy and repress red/far-red-light-reversible germination downstream of phytochrome B (phyB) in Arabidopsis thaliana . RVE1 and RVE2 expression is downregulated after imbibition and by phyB. RVE1 directly binds to the promoter of GIBBERELLIN 3-OXIDASE 2 , inhibits its transcription and thus suppresses the biosynthesis of bioactive gibberellins. In addition, DELAY OF GERMINATION 1 also acts downstream of phyB. This study identifies a signalling pathway that integrates environmental light input with internal factors to control both seed dormancy and germination. Seeds mediate the alternation of generations in flowering plants and have been a staple food throughout human civilization. Primary seed dormancy is acquired during seed maturation and reaches a high level in freshly harvested seeds and maintained for a certain period that allows seeds to survive under unfavourable conditions and prevents pre-harvest sprouting, and is thus an important aspect of plant fitness [1] , [2] , [3] . Under optimal conditions, the release of dormancy by after-ripening and the successful germination and establishment of a robust seedling are critical for the propagation of the plant species [4] , [5] . Dormancy and germination are two distinct but closely connected physiological processes. The dormancy-to-germination transition is a critical developmental step in the life cycle of plants that is determined by both genetic factors and environmental influences [2] , [3] , [4] . The phytohormones gibberellin (GA) and abscisic acid (ABA) primarily and antagonistically regulate the seed status; GA represses dormancy and promotes germination, whereas ABA has the opposite effects. The signalling pathways that GA and ABA control seed germination have been extensively studied [2] , [6] , [7] , [8] , [9] . Previous genetic analyses have revealed many regulators that affect the induction, maintenance and release of seed dormancy [2] , [3] . Studies of natural variation have identified multiple quantitative trait loci (QTL) that contribute to dormancy in wild populations of Arabidopsis thaliana and some crops [10] , [11] , [12] , [13] , [14] , [15] . Among them, DELAY OF GERMINATION 1 ( DOG1 ) is a major QTL in a recombinant inbred line population of Arabidopsis [10] , [16] . DOG1 protein levels in freshly harvested dry seeds strongly correlate with the time required for after-ripening [17] . A recent study showed that DOG1 regulates primary seed dormancy through a microRNA pathway [18] . However, the molecular function and regulation of DOG1 remain elusive. Light is a major environmental signal that oppositely modulates the levels of GA and ABA, and affects seed germination [8] , [19] , [20] . Among plant photoreceptors, the red and far-red-light-absorbing phytochromes are essential for light promotion of germination [21] . In the model species Arabidopsis , five genes ( PHYA to PHYE ) encode phytochrome apoproteins [22] , [23] . Phytochrome B (phyB) predominantly triggers red/far-red-light-reversible seed germination, whereas phyA mediates distinct, very low fluence responses in red and far-red light [24] , [25] , [26] , [27] , [28] , [29] , [30] , [31] . phyA- and phyB-dependent induction of germination are spatially separated in the endosperm and embryo [32] . phyE is required for germination in continuous far-red light [33] . A recent study shows that phyE and phyD stimulate germination at very low red/far-red ratios and, surprisingly, phyC antagonizes the promotion of germination by light [34] . At the molecular level, far-red light converts phyochromes into the inactive Pr form, which inhibits seed germination, whereas a subsequent red-light pulse reverts it to active Pfr and induces germination [22] , [35] . Light-activated phyB interacts with and promotes the degradation of a negative regulator, PHYTOCHROME-INTERACTING FACTOR 1 (PIF1, also known as PIL5) [36] , [37] . PIF1 directly regulates the expression of several downstream genes, including GA-INSENSITIVE , REPRESSOR OF GA1-3 and SOMNUS , which modulates GA responsiveness, GA and ABA biosynthesis and subsequent seed germination [38] , [39] , [40] , [41] . PIF6 was previously shown to regulate the primary seed dormancy [42] . Although phytochromes are involved in regulating seed dormancy [21] , [28] , [43] , the underlying molecular mechanism was hitherto unknown. REVEILLE1 (RVE1) belongs to a subfamily of Myb-like transcription factors that includes CIRCADIAN CLOCK-ASSOCIATED 1 (CCA1) and LATE ELONGATED HYPOCOTYL clock components [44] , [45] . RVE1 regulates hypocotyl growth by integrating the circadian clock and auxin pathways [44] . We previously revealed that RVE1 modulates chlorophyll biosynthesis and seedling de-etiolation in Arabidopsis [46] . In this study, we identified RVE1 and RVE2 as activators of seed dormancy and further provided molecular and genetic evidence to show that RVE1 and RVE2 promote primary seed dormancy and repress red/far-red-light-mediated germination downstream of phyB in A. thaliana . We found that the transcription of RVE1 , RVE2 and DOG1 is reduced by phyB-Pfr, the active form of phyB. We also demonstrate that RVE1 directly inhibits GIBBERELLIN 3-OXIDASE 2 ( GA3ox2 ) transcription and subsequently suppresses bioactive GA biosynthesis. Therefore, we reveal a genetic pathway that links light input with internal factors to control seed dormancy and germination that can potentially optimize seed adaptability to changing environments. RVE1 and RVE2 regulate seed dormancy and germination We first examined the role of RVE1 in light-induced seed germination using 2- to 5-month post-harvest seeds. The after-ripening seeds were exposed to different light conditions without cold stratification ( Fig. 1a ). The phyB photoreceptor positively controls red/far-red reversible seed germination [25] , [26] , [27] . As shown in Fig. 1b,c , under phyB-off conditions (grown in darkness interrupted by a 5-min pulse of far-red light to inactivate phyB), Columbia (Col) wild-type seeds did not germinate, whereas the germination frequency of rve1 -null mutant ( Supplementary Fig. 1a,b ) was close to 40%. Under darkness or phyB-on conditions (grown in darkness interrupted by a 5-min pulse of far-red light followed by 5-min pulse of red light to activate phyB), 100% of the rve1 seeds germinated, similar to Col. Remarkably, RVE1 overexpression ( RVE1-OX ) transgenic seeds failed to germinate under all conditions ( Fig. 1b,c ). It was further supported by a time-course germination assay ( Supplementary Fig. 1c ). The pif1 seeds, which were used as a control, germinated under all conditions tested, as reported previously ( Fig. 1b,c ) [38] . These observations suggest that RVE1 negatively regulates phyB-mediated seed germination. 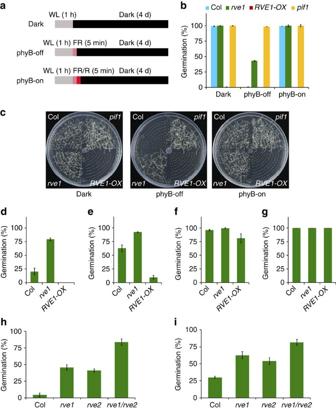Figure 1: RVE1 regulates both seed dormancy and germination. (a) Light irradiation treatment in the experiments. Post-harvest seeds were irradiated with white light (WL) for 1 h (starting from seed sterilization) and were then exposed to far-red (FR) light for 5 min (phyB-off) or followed by 5 min of red (R) light (phyB-on). Seeds were then kept in darkness and germination frequencies were recorded after 4 days. (b) Quantification of the germination frequencies of seeds under different conditions as shown ina. (c) Representative images of seed germination assays of Col,rve1andRVE1-OXseeds under the light conditions shown ina. (d–g) Percentage of seed germination. Freshly harvested seeds were kept in darkness (d) or under white light (e) for 3 days, or seeds were stratified at 4 °C for 1 day (f) or 3 days (g) in darkness before being exposed to 3 days of white light treatment at 22 °C. (h) Germination percentage of post-harvest seeds ofrve1,rve2andrve1/rve2grown under the phyB-off condition. (i) Dormancy phenotype of freshly harvested seeds ofrve1,rve2andrve1/rve2grown in darkness for 4 days. Forbandd–i, mean±s.d.,n=3. Figure 1: RVE1 regulates both seed dormancy and germination. ( a ) Light irradiation treatment in the experiments. Post-harvest seeds were irradiated with white light (WL) for 1 h (starting from seed sterilization) and were then exposed to far-red (FR) light for 5 min (phyB-off) or followed by 5 min of red (R) light (phyB-on). Seeds were then kept in darkness and germination frequencies were recorded after 4 days. ( b ) Quantification of the germination frequencies of seeds under different conditions as shown in a . ( c ) Representative images of seed germination assays of Col, rve1 and RVE1-OX seeds under the light conditions shown in a . ( d – g ) Percentage of seed germination. Freshly harvested seeds were kept in darkness ( d ) or under white light ( e ) for 3 days, or seeds were stratified at 4 °C for 1 day ( f ) or 3 days ( g ) in darkness before being exposed to 3 days of white light treatment at 22 °C. ( h ) Germination percentage of post-harvest seeds of rve1 , rve2 and rve1/rve2 grown under the phyB-off condition. ( i ) Dormancy phenotype of freshly harvested seeds of rve1 , rve2 and rve1/rve2 grown in darkness for 4 days. For b and d – i , mean±s.d., n =3. Full size image Next, we asked whether RVE1 is involved in seed dormancy using freshly harvested seeds. We found that ∼ 80% of the rve1 seeds germinated compared with ∼ 20% of Col seeds, whereas RVE1-OX seeds failed to germinate in dark condition ( Fig. 1d ). Under white light conditions, ∼ 60% of Col seeds germinated, whereas ∼ 90% of rve1 seeds and <10% of RVE1-OX seeds germinated ( Fig. 1e ). Notably, after 1 day of cold stratification followed by 3 days of exposure to white light treatment at 22 °C, almost all Col seeds germinated, whereas ∼ 80% of RVE1-OX seeds germinated ( Fig. 1f ). This reduced germination rate was not due to developmental defects, because all of the RVE1-OX seeds germinated after 3 days of cold stratification ( Fig. 1g ). In addition, a far-red light pulse (phyB-off) inhibited germination of rve1 , whereas a further red light pulse induced germination of freshly harvested seeds ( Supplementary Fig. 1d ). Another line of RVE1 overexpression plant ( 35S:Myc-RVE1 ) showed a similar response to RVE1-OX ( Supplementary Fig. 1e ). RVE2 is the closest homolog of RVE1 (ref. 47 ). Similar to rve1 , rve2 -null mutant seeds displayed increased seed germination ( Supplementary Fig. 2 ) and the rve1/rve2 double mutant had even higher germination frequencies than the single mutants ( Fig. 1h,i ). Overexpression of RVE2 ( RVE2-OX ) resulted in reduced phyB-mediated seed germination ( Supplementary Fig. 2c ). RVE2-OX also conferred the dormancy response ( Supplementary Fig. 2d ). Taken together, these phenotypic analyses indicate that RVE1 and RVE2 play additive and dual roles in controlling both primary seed dormancy and phyB-dependent seed germination. RVE1 and DOG1 act genetically downstream of phyB Early studies suggest the involvement of phyB in seed germination of freshly harvested seeds [21] , [28] . We further observed that freshly harvested phyB mutant seeds exhibited a strong dormant phenotype under white light ( Fig. 2a ), whereas two lines of PHYB overexpression transgenic seeds, 35S:Myc-PHYB ( Supplementary Fig. 3a ) and PHYB-ABO , had a greater germination frequency than their corresponding wild-type controls in darkness ( Fig. 2b,c ). Interestingly, PHYB overexpression seeds had 100% germination frequencies compared with 30–35% for wild-type seeds under complete darkness ( Supplementary Fig. 3b ). These data confirm that phyB suppresses primary seed dormancy. We then generated a rve1/phyB double mutant by genetic crossing between rve1 and phyB-9 . The reduced dormancy of rve1 was partly suppressed by phyB mutation in the rve1/phyB double mutant ( Fig. 2a ). Moreover, the post-harvest phyB seeds had low germination rates in darkness ( Fig. 2d ). Notably, homozygous rve1/phyB had germination frequencies close to those of rve1 under all conditions ( Fig. 2d ). These results suggest that RVE1 acts genetically downstream of phyB to regulate primary seed dormancy and red/far-red light reversible germination. 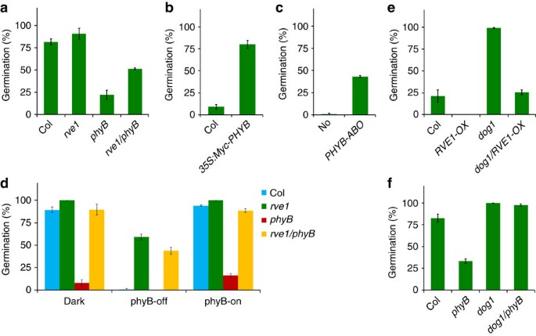Figure 2: Genetic interaction with phyB. (a) Germination frequency of freshly harvested seeds of Col,phyB-9,rve1andrve1/phyBincubated under white light for 4 days. (b) Germination frequency of freshly harvested Col wild-type and35S:Myc-PHYBtransgenic seeds incubated in darkness for 4 days. (c) Germination frequency of freshly harvested Nossen (No)-0 wild-type andPHYB-ABOtransgenic seeds incubated in darkness for 4 days. (d) Germination frequency of post-harvest seeds of Col,phyB-9,rve1andrve1/phyBincubated under different light conditions as indicated inFig. 1a. (e) Seed dormancy response of freshly harvested seeds of Col,RVE1-OX,dog1anddog1/RVE1-OXgrown in darkness for 4 days. (f) Dormancy response of freshly harvested seeds of Col,phyB,dog1anddog1/phyBincubated under white light for 4 days. Fora–f, mean±s.d.,n=3. Figure 2: Genetic interaction with phyB. ( a ) Germination frequency of freshly harvested seeds of Col, phyB-9 , rve1 and rve1/phyB incubated under white light for 4 days. ( b ) Germination frequency of freshly harvested Col wild-type and 35S:Myc-PHYB transgenic seeds incubated in darkness for 4 days. ( c ) Germination frequency of freshly harvested Nossen (No)-0 wild-type and PHYB-ABO transgenic seeds incubated in darkness for 4 days. ( d ) Germination frequency of post-harvest seeds of Col, phyB-9 , rve1 and rve1/phyB incubated under different light conditions as indicated in Fig. 1a . ( e ) Seed dormancy response of freshly harvested seeds of Col, RVE1-OX , dog1 and dog1 / RVE1-OX grown in darkness for 4 days. ( f ) Dormancy response of freshly harvested seeds of Col, phyB , dog1 and dog1/phyB incubated under white light for 4 days. For a – f , mean±s.d., n =3. Full size image DOG1 is an important suppressor of seed dormancy [16] , [17] , [18] . To examine the relationship between RVE1 and DOG1, we introduced RVE1-OX into the dog1 -null mutant background. Overexpression of RVE1 complemented the non-dormant phenotype of dog1 in the dog1/RVE1-OX homozygous seeds in darkness ( Fig. 2e ). Furthermore, DOG1 acted downstream of phyB in the regulation of primary seed dormancy ( Fig. 2f ). RVE1/2 and DOG1 expression is inhibited by phyB Next, we evaluated the expression pattern of RVE1 , RVE2 and DOG1 during embryogenesis from public data repositories [48] . The transcript levels of RVE1 , RVE2 and DOG1 increase gradually during seed development ( Supplementary Fig. 4 and ref. 17 ), indicating that they are required for dormancy induction. However, the other RVE genes and PIF1 did not display such an expression mode ( Supplementary Fig. 4 ). Quantitative reverse transcriptase–PCR showed that, similar to DOG1 , RVE1 and RVE2 expression was rapidly decreased in freshly harvested wild-type seeds during imbibition ( Fig. 3a ) [17] . We next examined whether the expression of RVE1 and RVE2 correlates with the level of dormancy in different ecotypes. Under white light, freshly harvested seeds of Col and Landsberg erecta accessions were non-dormant and those of Wassilewskija and Köln ecotypes were partially dormant, whereas Cape Verde Island seeds were completely dormant ( Fig. 3b ). Conversely, the level of RVE1 and RVE2 transcripts increased with the degree of dormancy of these ecotypes ( Fig. 3c ). Furthermore, the expression of RVE1 , RVE2 and DOG1 was drastically reduced by a red light pulse (phyB-on) in Col seeds ( Fig. 3d ). We then generated RVE1p:GUS transgenic plants in which β-glucuronidase (GUS) reporter expression was driven by the RVE1 promoter sequence (1.4 kb upstream of the ATG start codon). Under phyB-off condition, the cotyledons and radical of RVE1p:GUS seeds were stained in blue, whereas staining was greatly reduced under phyB-on conditions ( Fig. 3e ). RVE1p:GUS was also introduced into the phyB mutant. GUS expression in both the embryo and endosperm of fresh seeds was remarkably increased in phyB compared with in Col control ( Fig. 3f ). Consistently, the transcript levels of RVE1 , RVE2 and DOG1 were increased in phyB ( Fig. 3g ). However, a chromatin co-immunoprecipitation (ChIP) assay showed that phyB was not recruited to the chromatin of RVE1 , RVE2 and DOG1 genes ( Supplementary Fig. 5 ). These experiments confirm that RVE1 , RVE2 and DOG1 expression are repressed after imbibition and by active form of phyB. 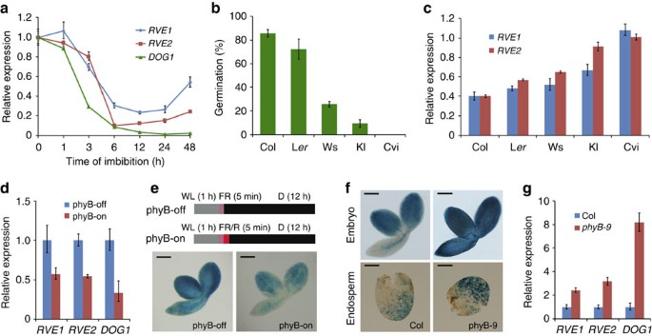Figure 3: Expression pattern ofRVE1andRVE2. (a) Relative expression ofRVE1,RVE2andDOG1during imbibition. Freshly harvested Col seeds were imbibed in 0.6% agar plates for the indicated time. (b) Germination frequency of freshly harvested seeds from Col, Landsbergerecta(Ler), Wassilewskija (Ws), Köln (Kl) and Cape Verde Islands (Cvi) ecotypes. Seeds were grown under white light conditions for 4 days. (c) Relative expression levels ofRVE1andRVE2in different ecotypes. Total RNA was isolated from seeds imbibed under light for 12 h. (d) Quantitative reverse transcriptase–PCR ofRVE1andRVE2in post-harvest Col seeds grown under phyB-off and phyB-on conditions. (e) GUS staining ofRVE1p:GUStransgenic seeds after phyB-off and phyB-on treatments as indicated in the top panels. D, dark; FR, far-red light; R, red light; WL, white light. (f) GUS staining of freshly harvested Col andphyBseeds harbouringRVE1p:GUS.The seeds were incubated in darkness for 12 h. Scale bars, 200 μm (e,f). (g) Relative expression ofRVE1,RVE2andDOG1in Col and thephyB-9mutant. Freshly harvested seeds were imbibed for 36 h in darkness. Fora–dandg, mean±s.d.,n=3. Figure 3: Expression pattern of RVE1 and RVE2 . ( a ) Relative expression of RVE1 , RVE2 and DOG1 during imbibition. Freshly harvested Col seeds were imbibed in 0.6% agar plates for the indicated time. ( b ) Germination frequency of freshly harvested seeds from Col, Landsberg erecta (L er ), Wassilewskija (Ws), Köln (Kl) and Cape Verde Islands (Cvi) ecotypes. Seeds were grown under white light conditions for 4 days. ( c ) Relative expression levels of RVE1 and RVE2 in different ecotypes. Total RNA was isolated from seeds imbibed under light for 12 h. ( d ) Quantitative reverse transcriptase–PCR of RVE1 and RVE2 in post-harvest Col seeds grown under phyB-off and phyB-on conditions. ( e ) GUS staining of RVE1p:GUS transgenic seeds after phyB-off and phyB-on treatments as indicated in the top panels. D, dark; FR, far-red light; R, red light; WL, white light. ( f ) GUS staining of freshly harvested Col and phyB seeds harbouring RVE1p:GUS. The seeds were incubated in darkness for 12 h. Scale bars, 200 μm ( e , f ). ( g ) Relative expression of RVE1 , RVE2 and DOG1 in Col and the phyB-9 mutant. Freshly harvested seeds were imbibed for 36 h in darkness. For a – d and g , mean±s.d., n =3. Full size image RVE1 directly and specifically represses GA3ox2 expression Seed dormancy and germination are predominantly regulated by the balance of GA and ABA levels [2] , [7] , [8] . To reveal the molecular mechanism underlying RVE1 function, we examined the expression of most metabolic genes of the GA and ABA biosynthetic pathways between Col and RVE1-OX seeds grown under phyB-on conditions. The GA biosynthetic pathway is catalysed by GA 20-oxidase and GA 3-oxidase (GA3ox) to produce bioactive hormones, which are subsequently deactivated by multiple classes of enzymes such as GA 2-oxidase [49] . ABA is a sesquiterpenoid derived from carotenoids by a series of enzymes [50] . The expression levels of several ABA metabolic genes, including ABA-DEFICIENT 1 ( ABA1 ), ABA3 , NINE-CIS-EPOXYCAROTENOID DEOXYGENASE 5 and CYTOCHROME P450 FAMILY 707 SUBFAMILY A POLYPEPTIDE 2 in RVE1-OX were about 1.5- to 2-fold of those in Col, whereas the transcript levels of ABA4 , CYP707A3 and two GA metabolic genes, GA20ox1 and GA3ox1 , were decreased in RVE1-OX by 1- to 2-fold as compared with Col ( Fig. 4a and Supplementary Fig. 6 ). Most remarkably, GA3ox2 expression was drastically decreased by ∼ 13-fold in RVE1-OX seeds ( Fig. 4a ). These analyses suggest that RVE1 regulates the expression of both ABA and GA biosynthetic genes. 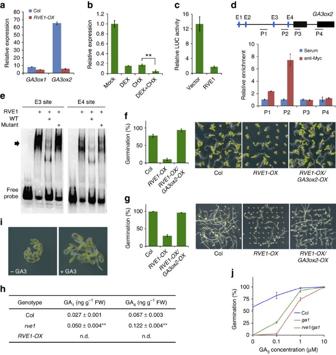Figure 4: RVE1 regulates GA biosynthesis by directly modulatingGA3ox2expression. (a) Relative expression levels ofGA3ox1andGA3ox2in Col andRVE1-OXgrown under phyB-on conditions. (b) Relative expression levels ofGA3ox2in35S:RVE1-GRtransgenic seeds incubated in darkness for 24 h without (Mock, 0.05% dimethy; sulfoxide (DMSO)) or with 5 μM DEX and/or 50 μM cycloheximide (CHX). Asterisks denote statistically significant difference (P<0.01, Student’st-test). (c) Transient transcriptional assay ofGA3ox2p:LUCbyRVE1overexpression or empty vector control inArabidopsisprotoplasts. (d) ChIP assay ofGA3ox2DNA precipitated in35S:Myc-RVE1by Myc antibody or serum control. Post-harvested35S:Myc-RVE1seeds were incubated under phyB-on condition. The top diagram indicates the genomic structure ofGA3ox2. Black boxes indicate exons. P1 to P4 fragments show PCR regions in the ChIP assay and E1 to E4 sites are putative EE-expand motifs. (e) EMSA assay. The oligos were synthesized by fusing three copies of the E3 or E4 motifs and their flanking sequences. The oligos labelled with biotin were used for probes and incubated with or without RVE1 recombinant proteins. Excess amounts (× 50) of unlabelled wild-type (WT) or mutant oligos were added as the competitors. Arrow denotes shifted bands of protein–DNA complexes. (f) Seed dormancy phenotype of Col,RVE1-OXandRVE1-OX/GA3ox2-OXtransgenic seeds grown under white light for 4 days. (g) Light-mediated seed germination phenotype of Col,RVE1-OXandRVE1-OX/GA3ox2-OXtransgenic seeds grown under phyB-on conditions. (h) Measurement of GA1and GA4contents of freshly harvested Col,rve1andRVE1-OXseeds imbibed in darkness for 24 h. Data are means±s.d.,n=3. n.d., not detected. Asterisks indicate significant differences from Col using Student’st-test (P<0.01). (i) Germination phenotype ofRVE1-OXin the absence or presence of exogenous GA3(10 μM). Seed coats were removed to facilitate GA3absorption and embryos were incubated in darkness for 2 days. (j) Germination percentage of Col,ga1andrve1/ga1in the absence or presence of various concentrations of exogenous GA3. Freshly harvested seeds were incubated under white light for 3 days. For all column figures, mean±s.d.,n=3. Figure 4: RVE1 regulates GA biosynthesis by directly modulating GA3ox2 expression. ( a ) Relative expression levels of GA3ox1 and GA3ox2 in Col and RVE1-OX grown under phyB-on conditions. ( b ) Relative expression levels of GA3ox2 in 35S:RVE1-GR transgenic seeds incubated in darkness for 24 h without (Mock, 0.05% dimethy; sulfoxide (DMSO)) or with 5 μM DEX and/or 50 μM cycloheximide (CHX). Asterisks denote statistically significant difference ( P <0.01, Student’s t -test). ( c ) Transient transcriptional assay of GA3ox2p:LUC by RVE1 overexpression or empty vector control in Arabidopsis protoplasts. ( d ) ChIP assay of GA3ox2 DNA precipitated in 35S:Myc-RVE1 by Myc antibody or serum control. Post-harvested 35S:Myc-RVE1 seeds were incubated under phyB-on condition. The top diagram indicates the genomic structure of GA3ox2 . Black boxes indicate exons. P1 to P4 fragments show PCR regions in the ChIP assay and E1 to E4 sites are putative EE-expand motifs. ( e ) EMSA assay. The oligos were synthesized by fusing three copies of the E3 or E4 motifs and their flanking sequences. The oligos labelled with biotin were used for probes and incubated with or without RVE1 recombinant proteins. Excess amounts (× 50) of unlabelled wild-type (WT) or mutant oligos were added as the competitors. Arrow denotes shifted bands of protein–DNA complexes. ( f ) Seed dormancy phenotype of Col, RVE1-OX and RVE1-OX / GA3ox2-OX transgenic seeds grown under white light for 4 days. ( g ) Light-mediated seed germination phenotype of Col, RVE1-OX and RVE1-OX / GA3ox2-OX transgenic seeds grown under phyB-on conditions. ( h ) Measurement of GA 1 and GA 4 contents of freshly harvested Col, rve1 and RVE1-OX seeds imbibed in darkness for 24 h. Data are means±s.d., n =3. n.d., not detected. Asterisks indicate significant differences from Col using Student’s t -test ( P <0.01). ( i ) Germination phenotype of RVE1-OX in the absence or presence of exogenous GA 3 (10 μM). Seed coats were removed to facilitate GA 3 absorption and embryos were incubated in darkness for 2 days. ( j ) Germination percentage of Col, ga1 and rve1/ga1 in the absence or presence of various concentrations of exogenous GA 3 . Freshly harvested seeds were incubated under white light for 3 days. For all column figures, mean±s.d., n =3. Full size image To test whether RVE1 directly regulates the expression of these genes, we generated 35S:RVE1-GR transgenic lines in which RVE1 is fused to a sequence encoding the steroid-binding domain of the rat glucocorticoid receptor (GR) to control its nuclear translocation. In the presence of the glucocorticoid hormone dexamethasone (DEX), 35S:RVE1-GR showed the long hypocotyl phenotype, as did RVE1-OX ( Supplementary Fig. 7a ). With or without cycloheximide, a reagent that blocks protein synthesis, DEX treatment caused the transcript level of GA3ox2 , but not of the other GA and ABA metabolic genes tested, to drastically decrease ( Fig. 4b and Supplementary Fig. 7b ), suggesting that repression of GA3ox2 requires nuclear targeting of RVE1. Next, we carried out a transient expression assay in Arabidopsis mesophyll protoplasts and found that RVE1 greatly repressed the expression of the luciferase (LUC) reporter gene driven by the GA3ox2 promoter ( Fig. 4c ). In agreement with this observation, RVE1 possesses transcriptional repression activity ( Supplementary Fig. 8 ). To confirm the direct effect of RVE1 on GA3ox2 transcription, we performed ChIP assay using 35S:Myc-RVE1 seeds and Myc antibody. In contrast to the serum control, the Myc antibody pulled down the P2 fragment and, to a less extent, of P1 fragment in the promoter region of GA3ox2 , but not of GA3ox1 , in samples prepared under phyB-on conditions ( Fig. 4d and Supplementary Fig. 9 ). CCA1 is occupied at DNA regions containing several conserved motifs, such as evening element (EE) and EE-expand sequences [51] . As RVE1 and CCA1 are in the same subfamily of Myb-like proteins [44] , we reasoned that RVE1 might also bind to target genes via these motifs. By analysing the promoter sequence of GA3ox2 , we found that there are four putative EE-expand motifs, sites E1 (5′-AGATATGA-3′) and E2 (5′-GGATATGT-3′) being upstream of P1 fragment, site E3 (5′-GATATTA-3′) locating between P1 and P2 fragment, and site E4 (5′-TCATATCA-3′) being adjacent to P2 fragment ( Fig. 4d ). E3 and E4 were most likely to be the binding sites of RVE1 based on the ChIP result. To test this possibility, we purified RVE1 recombinant protein and carried out an electrophoresis mobility shift assay (EMSA). As shown in Fig. 4e , incubation with RVE1 protein caused strong mobility shift bands of probes for both E3 and E4 sites. Most intriguingly, addition of excess unlabelled wild-type oligos significantly reduced the binding, whereas addition of mutant oligos (5′-GATATTA-3′ changed to 5′-gggATag-3′ in E3, and 5′-TCATATCA-3′ changed to 5′-cgtctcag-3′ in E4) did not affect the shift ( Fig. 4e ), indicating that RVE1 directly binds to the specific EE-expands motifs of GA3ox2 in vitro . These results together confirm that RVE1 directly represses GA3ox2 expression. RVE1 regulates GA biosynthesis Next, we constructed transgenic plants overexpressing GA3ox2 in the RVE1-OX background ( RVE1-OX/GA3ox2-OX ) and used the resulting homozygous seeds to examine the genetic relationship between GA3ox2 and RVE1 . Overexpression of GA3ox2 complemented both the dormancy and germination phenotypes of RVE1-OX in RVE1-OX/GA3ox2-OX ( Fig. 4f,g ), suggesting that GA3ox2 acts genetically downstream of RVE1 . GA3ox2 encodes a GA3ox, which catalyses the production of bioactive GAs [49] . We reasoned that the impaired expression of GA3ox2 in the RVE1 mutant or overexpression seeds would alter endogenous GA levels. As expected, the content of bioactive forms of GA, including GA 1 and GA 4 , nearly doubled in freshly harvested rve1 seeds, but were undetectable in RVE1-OX seeds, compared with the Col control ( Fig. 4h ). However, ABA levels in rve1 and rve1/rve2 were indistinguishable from those in the wild-type control ( Supplementary Fig. 10 ). We then asked whether exogenous application of GA 3 could rescue the RVE1-OX phenotype. As shown in Fig. 4i , GA 3 treatment indeed rescued germination of RVE1-OX seeds. GA biosynthetic mutants such as gibberellic acid-requiring1-3 , lacking synthesis of de novo GA due to a defect in an early step of the GA metabolic pathway, do not germinate even under favourable conditions [52] . The rve1/ga1 double mutant was unable to germinate, as was the ga1 single mutant, but germinated better than ga1 in the presence of exogenous GA 3 ( Fig. 4j ), suggesting that RVE1 function requires GA biosynthesis. Taken together, these data indicate that RVE1 indeed specifically controls GA biosynthesis through direct regulation of GA3ox2 and probably also of other genes in an indirect manner. Phytochrome-mediated red/far-red-light-reversible regulation on seed germination has been extensively studied and signalling pathways have been proposed [22] , [41] , [53] . The involvement of light in regulating primary seed dormancy was previously observed in phytochrome-deficient mutants [21] , [28] , [54] ; however, the underlying molecular mechanism is not understood. In this report, we used freshly harvested seeds to study primary dormancy and after-ripened seeds to determine germination, and identified RVE1 and RVE2 as two novel factors in regulating both processes by light. We show that RVE1 and RVE2 transcription factors function additively downstream of phyB in controlling primary seed dormancy and germination ( Figs 1 and 2 ), supporting the idea that dormancy is regulated by phytochromes [21] , [42] . Expression of RVE1 , RVE2 and DOG1 is increased during seed development probably to induce seed dormancy ( Supplementary Fig. 4 ) [17] . phyB apoprotein accumulates during seed maturation [25] and is activated after imbibition to repress RVE1 , RVE2 and DOG1 expression ( Fig. 3 ). Overexpressing PHYB breaks dormancy even under darkness, possibly due to seeds producing Pfr form of phyB in the maternal environment during maturation and its constitutive inhibition of the transcription of RVE1/2 and DOG1 . As phytochromes relay light signals to PIF proteins [22] , [35] and phyB is not able to associate with the DNA sequences of RVE1 , RVE2 and DOG1 ( Supplementary Fig. 5 ), phyB might inhibit their expression indirectly through PIF1 and PIF6 transcription factors. In agreement with this, PIF1 activates RVE1 and RVE2 transcription ( Supplementary Fig. 11a,b ). PIF1 acts as a key transcription factor in modulating far-red/red-light-reversible germination of post-harvest seeds [38] , [39] , [40] . However, PIF1 is not involved in regulating primary dormancy of freshly harvested seeds ( Supplementary Fig. 1f ) [42] . Conversely, an alternative splice form of PIF6 regulates primary seed dormancy, but not light-mediated seed germination [42] . Here we demonstrate that RVE1 and RVE2 control both the establishment of primary dormancy and red/far-red-light-reversible seed germination. Therefore, seed dormancy and germination are differentially regulated via overlap and distinct pathways by light. We reveal that, at the molecular level, RVE1 directly binds to the conserved motif of GA3ox2 , represses its expression and controls bioactive GA accumulation in imbibed seeds ( Fig. 4 ). Other GA biosynthetic genes, such as GA3ox1 , are indirectly regulated by RVE1. However, ABA level was not affected by RVE1 and RVE2, although the expression of some ABA catabolic genes was regulated by RVE1, suggesting that RVE1/RVE2 specifically control the GA biosynthetic pathway. Consistently, seed responsiveness to GA is mainly controlled by phyB [34] . Therefore, we identify a previously unexplored signalling pathway, consisting of the phyB photoreceptor, RVE1 and RVE2 transcription factors, and GA3ox2, which plays critical roles in regulating GA biosynthesis and eventually primary seed dormancy and light-dependent germination ( Fig. 5 ). As the rve1/rve2 seeds had ∼ 80% germination rate ( Fig. 1i ), other factors and/or signalling mechanisms could be involved in the control of dormancy by light. phyA acts differentially to phyB in promoting seed germination [29] , [31] , [32] . Strikingly, we found that RVE1 also negatively regulated phyA-dependent seed germination ( Supplementary Fig. 12 ). Moreover, RVE1 acts as a transcription factor that regulates different biological functions probably through directly controlling of the expression of downstream genes [46] . 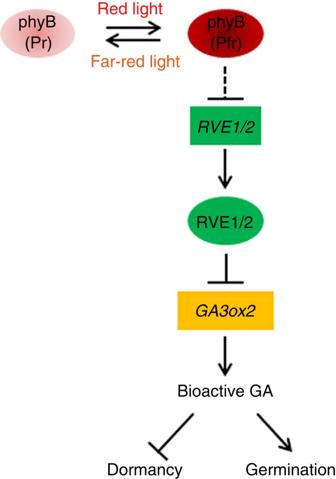Figure 5: A proposed working model of the phyB-RVE1/2 pathway in regulating seed dormancy and germination. During seed development, the transcripts ofRVE1andRVE2are increasingly accumulated to induce and maintain seeds at the dormant state. Red light triggers the activation of phyB (Pfr form), which repressesRVE1andRVE2expression, leading to the de-suppression of the GA biosynthetic geneGA3ox2and the accumulation of bioactive GAs, and consequently the induction of seed germination. Figure 5: A proposed working model of the phyB-RVE1/2 pathway in regulating seed dormancy and germination. During seed development, the transcripts of RVE1 and RVE2 are increasingly accumulated to induce and maintain seeds at the dormant state. Red light triggers the activation of phyB (Pfr form), which represses RVE1 and RVE2 expression, leading to the de-suppression of the GA biosynthetic gene GA3ox2 and the accumulation of bioactive GAs, and consequently the induction of seed germination. Full size image DOG1 is a key factor specific for the induction of primary seed dormancy [3] , [17] . Overexpression of RVE1 suppresses dog1 mutant phenotype and that DOG1 acts genetically downstream of phyB ( Fig. 2e,f ), suggesting that RVE1/RVE2 and DOG1 have similar roles, consistent with their similar expression patterns. Interestingly, RVE1 and DOG1 promote the transcription of each other ( Supplementary Fig. 11c,d ), although the regulatory mechanism requires further investigation. DOG1 protein levels predict the dormancy status of freshly harvested seeds [17] . It will be of interest to find out whether the proteins of RVE1 and RVE2 act similarly. Previous studies have identified seven QTLs for seed dormancy, three of which (that is, DOG1 , DOG4 and DOG7 ) are located on chromosome 5 in Arabidopsis [10] . Interestingly, RVE1 (At5g17300) and RVE2 (At5g37260) were located approximately within the genomic regions of DOG4 and DOG7 loci ( Supplementary Fig. 13 ), pointing to the possibility that RVE1 and RVE2 might correspond to DOG4 and DOG7 , respectively, and further arguing the importance of RVE1 and RVE2 in controlling seed dormancy. In supporting this proposition, RVE1 and RVE2 transcript levels positively correlate with the depth of dormancy in different ecotypes ( Fig. 3b,c ). Further genetic and molecular experiments are required to verify this possibility in the future. Light and temperature are two of the important environmental cues affecting seed dormancy and germination. Phytochromes appear to be involved in germination in response to photoperiod and temperature during seed development [54] . Specific phytochrome members contribute to germination differentially, depending on the temperature experienced by seeds during maturation and after dispersal; phyB is important to germination across a wide range of temperature [21] , [55] . It has been known that phytochromes control the expression of GA and ABA metabolic genes [8] , [20] , [32] . A recent study reveals that DOG1 mediates the temperature- and GA-dependent control of germination [56] . Moreover, RVE1 and RVE2 are homologues of the clock oscillator, CCA1, and RVE1 controls daily rhythms of auxin production by integrating the circadian and auxin signalling pathways [44] , [47] . Thus, phytochromes (such as phyB) and RVE1/RVE2 could integrate different environmental inputs (light, circadian and temperature) to modulate endogenous phytohormone metabolic and signalling pathways that control seed dormancy and germination [2] , [3] , [4] , which represents a common genetic adaptation mechanism to various habitats of seeds. Insufficient seed dormancy can lead to pre-harvest sprouting, whereas too much dormancy prevents uniform germination. Thus, optimal level of seed dormancy is an important agronomic trait for crops [57] . The light regulatory networks of seed dormancy and germination might be conserved in species that could help to improve plants’ fitness [3] , [58] . Plant materials and growth conditions The rve1-2 (SAIL_326_A01), rve2-1 (Salk_051843), phyB-9 (ref. 59 ), dog1-2 (ref. 16 ), ga1 (Salk_109115) and pif1-2 (ref. 60 ) mutants, and RVE1-OX [44] , 35S:Myc-RVE1 (ref. 46 ), RVE2-OX [47] , 35S:Myc-PHYB and PIF1-OX [38] transgenic plants are in the A. thaliana Col ecotype. PHYB-ABO [61] is in the Nossen ecotype. Double mutants/transgenic plants were generated by genetic crossing and homozygous lines were used. After sterilization, seeds were sown on 0.6% agar (pH 5.7) plates. GA 3 , DEX and cycloheximide were supplied in the agar medium as indicated in the text. Far-red and red light were supplied by light-emitting diode light sources and white light was supplied by cool white fluorescent lamps. Adult plants were grown in soil with regular irrigation at 22±2 °C, 60–70% humidity and under long-day (16 h light/8 h dark) conditions in a growth chamber, and seeds were harvested at the same time in each batch. Dormancy and germination assay For the seed dormancy assay, seeds were freshly harvested ∼ 4–5 weeks after fertilization and were surface sterilized and plated on 0.6% agar (pH 5.7) within an hour. Seeds were either stratified or not at 4 °C for 1 to 3 days and the seeds were then incubated in darkness or white light (80 μmol m −2 s −1 ) as indicated in the text. Seeds with a protruded radical were considered as germinated seeds. For light-mediated germination assays, harvested seeds were dry-stored in eppendorf tubes in the dark at room temperature for 2 to 5 months, as dry after-ripening is a common method used to relieve dormancy [3] , [7] . For phyB-dependent germination, seeds were exposed to weak white light for 1 h (including sterilization and plating) and incubated in darkness or irradiated with far-red light (3.5 μmol m −2 s −1 ) for 5 min to inactivate phyB (phyB-off), or followed by 5 min of red light (20 μmol m −2 s −1 ) to activate phyB (phyB-on). For phyA-dependent germination, sterilized and plated seeds were imbibed for 1 h and irradiated with far-red light for 5 min. After 48 h of dark incubation, the seeds were irradiated with far-red light for 12 h. All seeds were then incubated in darkness for 2 days and the germination frequency was determined [39] . At least 100 seeds were used for each genotype in each experiment and three replicates were performed for statistical analysis. All experiments were carried out at least three times with similar results and one representative result is shown. Plasmid construction For the transient expression assay, a 2.5 kb fragment upstream of the GA3ox2 translational start code was PCR amplified and inserted into the pEASY-Blunt vector (TransGen), generating pEASY-GA3ox2p. The promoter fragment was released from pEASY-GA3ox2p cut with KpnI and PstI, and ligated into the KpnI–PstI site of the pGreenII0800-LUC vector [62] , to generate GA3ox2p:LUC . The RVE1 open reading frame was released from pEASY-RVE1 (ref. 45 ), digested with EcoRI and SalI, and inserted into the EcoRI–SalI sites of pGAL4BD and pGAL4BD-VP16 (ref. 63 ) to generate BD-RVE1 and BD-RVE1-VP16, respectively. The RVE1 fragment was also inserted into the MfeI–XhoI sites of pUC18-3HA to produce 35S:RVE1. The RVE1 complementary DNA was re-amplified from pEASY-RVE1 plasmid and digested with NcoI and PmlI. The RVE1 gene was then inserted into the NcoI–PmlI sites of pCAMBIA1301 ( http://www.cambia.org/daisy/cambia/585 ) to generate pCAMBIA-35S-RVE1. A GR fragment was amplified and digested with SwaI and PmlI, and then ligated into the SwaI–PmlI sites of pCAMBIA-35S-RVE1, generating 35S:RVE1-GR. HIS-RVE1, BD-ERF3RD-VP16, GAL4:LUC and 35S:GUS were produced as described previously [46] , [63] . To obtain the open reading frame of GA3ox2 and PHYB , first-strand cDNA was reverse transcribed from total RNA extracted from Col wild-type seedlings using oligo(dT)18 primer. The GA3ox2 and PHYB fragments were amplified using high-fidelity Pfu DNA polymerase (Invitrogen) and cloned into pEASY, resulting in pEASY-GA3ox2 and pEASY-PHYB, respectively. pEASY-GA3ox2 was cut with EcoRI and SalI to release the GA3ox2 fragment, which was then ligated into the EcoRI–XhoI site of pRI101-GFP (Takara), giving rise to 35S:GA3ox2 . To facilitate follow-up cloning, two XhoI sites within phyB were mutagenized without changing the encoded amino acids, to generate pEASY-phyB-XhoIm. The pEASY-phyB-XhoIm plasmids were digested with MfeI and XhoI, and the released phyB fragment was inserted into the EcoRI–SalI site of pRI101-MYC, resulting in 35S:Myc-PHYB . To construct RVE1p:GUS , a fragment upstream of the translational start code of RVE1 was amplified by PCR and cloned into pEASY, resulting in pEASY-RVE1p. The pEASY-RVE1p plasmid was digested with EcoRI and SalI to release the RVE1 promoter, which was then ligated into the EcoRI–SalI sites of the pBI101-GUS vector to generate RVE1p:GUS . All amplified fragments were validated by sequencing. Primers used for plasmid construction are listed in Supplementary Table 1 . The binary constructs were electroporated into Agrobacterium tumefaciens strain GV3101 and then introduced into the wild type or rve1-2 mutant via the floral dip method [64] . Transgenic plants were selected on MS plates in the presence of 50 mg l −1 kanamycin or hygromycin. Homozygous lines were used in the experiments. Gene expression analysis Sample treatments were described in the respective figure legends. Total RNA was extracted from seeds using Universal Plant Total RNA Extraction Kit (BioTeke) and first-strand cDNA was synthesized using reverse transcriptase (Invitrogen). Quantitative PCR was carried out using the SYBR Premix ExTaq Kit (Takara) following the manufacturer’s instructions. Three technical replicates were performed for each sample and the expression levels were normalized to those of PP2A . Each experiment was performed at least three times with similar results and one representative result is shown. Primers are listed in Supplementary Table 1 . ChIP assay ChIP assay was carried out according to a previous method [65] . Briefly, the 35S:Myc-RVE1 , 35S:Myc-PHYB or Col seeds were treated under conditions as described in the text and samples were treated with 1% formaldehyde for protein–DNA cross-linking. The chromatin complexes were isolated and sonicated to shear DNA into ∼ 0.5–2 kb fragments. After spin at 4 °C for 5 min at 13,000 r.p.m., the chromatin supernatant was pre-cleared with salmon sperm-sheared DNA/protein A agarose beads and equally divided into three tubes. The first two tubes were incubated with anti-Myc antibody (1:1,000 dilution, Abcam, ab32) or serum control overnight at 4 °C with gentle agitation. The third tube was used as input control. The samples in first two tubes were incubated with protein A agarose beads for 2 h at 4 °C. The beads were pelleted by centrifugation for 2 min at 13,000 r.p.m. The cross-linked chromatins were eluted and reversed by incubating with 5 M NaCl at 65 °C overnight. The proteins were digested with 14 mg ml −1 proteinase K and the DNA fragments were recovered and quantified by quantitative PCR using primers spanning the promoter and coding regions of GA3ox1 , GA3ox2 , RVE1 , RVE2 , DOG1 and UBQ10 control. Electrophoresis mobility shift assay HIS-RVE1 recombinant proteins were expressed in Escherichia coli BL21 (DE3) strain and purified using Ni-NTA Agraose (Qiagen). EMSA assay was performed using LightShift Chemiluminescent EMSA Kit (Pierce) according to the manufacturer’s protocol. The two complementary oligonucleotides were annealed and labelled with biotin and then incubated with HIS-RVE1 fusion proteins in the absence or presence of excess amounts of unlabelled wild-type or mutant oligonucleotides. The protein–DNA samples were then separated on 5% polyacrylamide gels and signal was captured with a Chemiluminescence Imaging system (Biostep). The oligonucleotides sequences are shown in Supplementary Table 1 . GUS histochemical analysis The RVE1p:GUS homozygous transgenic seeds were subjected to various light conditions as indicated in the text. The embryo and endosperm were dissected under a stereomicroscope (Olympus) in green light. The samples were incubated in 0.1 M sodium phosphate buffer containing 50 mM K 3 Fe(CN) 6 , 50 mM K 4 Fe(CN) 6 and 1 mM 5-bromo-4-chloro-3-indolyl-β- D -glucuronide at 37 °C for 3–6 h. GUS staining was examined under a stereomicroscope and images were captured by a digital camera (Olympus). GA and ABA content determination Freshly harvested seeds were imbibed in darkness for 24 h before sampling. For GA determination, seeds were weighted and ground to fine powder in liquid nitrogen. Internal standards of 1 ng g −1 2 H 2 -GA 1 and 1 ng g −1 2 H 2 -GA 4 were added to the samples followed by extraction with 500 μl solvent (methanol/H 2 O, 80/20, v/v) at 4 °C for 12 h. The supernatants were sequentially passed through the pre-conditioned tandem solid-phase extraction cartridges containing C 18 adsorbent (50 mg) and strong anion exchange adsorbent (200 mg). The strong anion exchange cartridge was then rinsed with 2 ml of 20% methanol (v/v) and the targeted acidic phytohormones were eluted by 3 ml acetonitrile with 1% formic acid (v/v). The eluent was evaporated under mild liquid nitrogen stream at 35 °C and re-dissolved in 100 μl H 2 O. The solution was acidified with 10 μl formic acid and extracted with 1 ml ether twice. The combined ether phase was dried under nitrogen gas and reconstituted in 100 μl acetonitrile followed by addition of 10 μl triethylamine (20 μmol ml −1 ) and 10 μl 3-bromoactonyltrimethylammonium bromide (20 μmol ml −1 ). The reaction solution was vortexed at 35 °C for 30 min and then evaporated under nitrogen gas. The samples were dissolved in 200 μl 10% acetonitrile (v/v) and subjected for Nano-liquid chromatography–electrospray ionization–quadrupole time-of-flight–mass spectrometry analysis [66] . For ABA measurement, seeds were ground in liquid nitrogen and 45 pmol of 2 H 2 -ABA internal standard was added to 200 mg of powder. The samples were extracted with 2 ml methanol at −20 °C overnight. After spin at 4 °C for 15 min at 18,000 r.p.m., the supernatant was dried under nitrogen gas and dissolved in 1 ml 5% ammonia solution (v/v). The crude extracts were purified by pre-conditioned Oasis MAX strong anion-exchange column (Waters) and the samples were eluted with 4 ml methanol containing 5% formic acid. The eluent was dried under nitrogen gas and dissolved in 200 μl 80% methanol (v/v) and subjected for ultra-performance liquid chromatography tandem mass spectrometry analysis [67] . LUC transient expression assay For transient expression of GA3ox2 by RVE1, the reporter plasmid GA3ox2p:LUC and 35S:RVE1 effector or vector control were co-transformed into Arabidopsis protoplasts. The protoplasts were pelleted and resuspended in 100 μl of × 1 cell culture lysis reagent (Promega). Luminescence activities of firefly and Renilla were measured using Dual-Luciferase Reporter Assay System reagent in a Modulus Luminometer/Fluorometer equipped with a luminescence kit (Promega). Five microlitres of the extract was first mixed with 15 μl of LAR II reagent to determine firefly luminescence (LUC firefly ). Fifteen microlitres of Stop and Glo assay reagent was then added to measure the Renilla luminescence (LUC Renilla ). The relative reporter expression level was expressed as the LUC firefly /LUC Renilla ratio. For RVE1 transcriptional activation activity assay, the reporter plasmid GAL4p:LUC, effector constructs (DB-RVE1, DB-VP16, DB-RVE1-VP16, DB-ERF3RD-VP16 or empty vector) and 35S:GUS internal control were co-transformed into Arabidopsis protoplasts. After cell lysis, 5 μl of the extract was mixed with 15 μl of LUC Assay Substrate (Promega) to determine LUC activity. For GUS enzymatic assay, 5 μl of the extract was incubated with 45 μl 4-methylumbelliferyl β- D -glucuronide assay buffer (50 mM sodium phosphate pH 7.0, 1 mM 4-methylumbelliferyl β- D -glucuronide, 10 mM EDTA, 10 mM β-mercaptoethanol, 0.1% sarkosyl and 0.1% Triton X-100) at 37 °C for 15 min and the reaction was stopped by adding 950 μl of 0.2 M Na 2 CO 3 . GUS fluorescence was measured using an ultraviolet fluorescence optical kit. The relative reporter expression level was expressed as the LUC/GUS ratios. Data availability The authors declare that all data supporting the findings of this study are available in the manuscript and its Supplementary Information files or are available from the corresponding author upon request. How to cite this article: Jiang, Z. et al. Phytochrome B and REVEILLE1/2-mediated signalling controls seed dormancy and germination in Arabidopsis . Nat. Commun. 7:12377 doi: 10.1038/ncomms12377 (2016).